Metallodendrimers in three oxidation states with electronically interacting metals and stabilization of size-selected gold nanoparticles Metallodendrimers containing redox-robust centres may have applications in molecular redox recognition, sensing, biosensing and catalysis. So far, however, no metallodendrimer is known in several oxidation states. Here we report metallodendrimers with two electronically communicating iron centres that are stable and isolated in both the Fe II and Fe III oxidation states, and in addition as class-II mixed-valent Fe II Fe III complexes. These dendrons are branched to arene-centred dendrimer cores either by Sonogashira coupling or ‘click’ reactions. The latter reaction involves the introduction of intradendritic 1,2,3-triazolyl ligands, which allows investigation of the selective role of these ligands in intradendritic Au III coordination and Au 0 nanoparticle stabilization. As a result, and using the various metallodendrimers with different oxidation states, small Au 0 nanoparticles are intradendritically stabilized by the triazole ligands, whereas with the related non-‘click’ dendrimers large Au 0 nanoparticles are formed outside the dendrimers and stabilized by a group of dendrimers. To date, dendrimers and metal nanoparticles (NPs) have been largely involved in materials science including nanomedicine, photonics and supramolecular chemistry [1] , [2] , [3] , [4] , [5] , and in particular metallodendrimers and dendrimer-containing NPs [2] , [3] , [4] , [6] , [7] , [8] , [9] , [10] , [11] have been efficiently designed for catalysis [2] , [3] , [4] , photophysics [7] , [8] , [9] , [10] , [11] and sensing [9] , [10] , [11] , [12] , [13] . Redox-stable metallodendrimers are a specific class of materials allowing redox anion recognition, sensing [2] , [3] , [4] , [5] , [6] , [7] , [8] , [9] , [10] , [11] , [12] , [13] , [14] , [15] , [16] and biosensing [14] , [15] that have been used essentially with ferrocene derivatives [12] , [13] , [14] , [15] . Although biferrocene- and silicon-bridged biferrocene-terminated dendrimers are known [5] , [14] , [15] , [16] , no dendrimers have yet been isolated in several oxidation states owing to instability of the odd-electron species. The flexibility of oxidation-state variation with the maintenance of stability for a large collection of metal centres located at the metallodendrimer periphery is highly desirable, however, because it would allow the design of nanodevices towards applications in molecular nanoelectronics including nanobatteries [17] and polyelectrolytes [18] . Here we present the synthesis and redox, electronic and NP-stabilization properties of new metallodendrimers in three robust oxidation states including mixed-valent metallodendrimers. The metal centres located at the dendritic periphery are organized in dendrons in such a way that the two metal centres of the dendrons are electronically communicating. Redox reactions of transition-metal complexes [19] , [20] , [21] , [22] are essential to organize molecular electronic communication in nanomaterials [23] . The redox-rich iron centres in the chosen system are Cp*Fe II (dppe)-alkynyl units (Cp*=η 5 -C 5 Me 5 , dppe=1,2-bis(diphenylphosphino)ethane) [24] that are isolobal to ferrocene and linked in meta position of an aryl bridge. In 1,3,5-trimetallaalkynylbenzene derivatives [24] , [25] , [26] , [27] , and in such Cp*Fe II (dppe) derivatives in particular [25] , [26] , it has been shown by density functional theory calculation and electrochemistry that, unlike in the 1,3,5-triferrocenylalkynylbenzene derivatives [28] , the three metals are electronically communicating. We synthesize the dendrons with only two iron-ethynyl groups in 1,3 position, leaving the third ethynyl position free for binding to the dendritic core either by Sonogashira coupling [29] , [30] or copper-catalysed azide-alkyne cycloaddition (CuAAC, ‘click’) reactions [31] , [32] , [33] with appropriately functionalized dendritic core termini. In this way, metallodendrimers in the three oxidation states Fe II Fe II , Fe II Fe III and Fe III Fe III are synthetically accessible with and without 1,2,3-triazolyl ligands on the branches, and the latter parameter strongly influences their ability to stabilize and isolate gold NPs (AuNPs) on HAuCl 4 reduction. As a result, we demonstrate how the presence and number of these intradendritic ligands is crucial to form well-defined, very small AuNPs. Dendron and dendrimer synthesis Both new bimetallic dendrons 1 and 2 were prepared from the precursor complex [FeCp*(dppe)Cl] according to Fig. 1 . Treatment of one equiv. of 1,3,5-triethynylbenzene with two equiv. of [FeCp*(dppe)Cl] and NH 4 PF 6 in a methanol/tetrahydrofuran (THF) mixture (1:1), followed by deprotonation with KOBu t produced 1-ethynyl-3,5-bis(iron)alkynylbenzene, 1 , with 60% yield, and 1-bromo-3,5-bis(iron)alkynylbenzene, 2 , was obtained upon reaction of [FeCp*(dppe)Cl] with 1-bromo-3,5-bis(ethynyl)benzene in 70% yield ( Fig. 1 ). Both complexes 1 and 2 were isolated as orange microcrystals following standard column chromatography. The characterizations of complexes 1 and 2 are gathered, respectively, in the Supplementary Figs 1–6 and 7–12 . 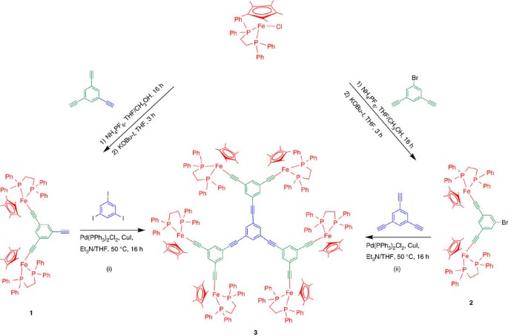Figure 1: Synthesis of dendrons and dendrimer 3. Reactions of [FeCp*(dppe)Cl] in the presence of NH4PF6with 1,3,5-triethynylbenzene and with 1-bromo-3,5-bis(ethynyl)benzene, both followed by deprotonation with KOBut, produced respectively the dendrons1and2. The hexanuclear compound3was obtained in two methods under Sonogashira reactions: (i) Sonogashira reaction between dendron1and 1,3,5-triiodobenzene catalysed by Pd(PPh3)2Cl2and CuI and (ii) reaction of dendron2with 1,3,5-triethynylbenzene under the same conditions. Figure 1: Synthesis of dendrons and dendrimer 3. Reactions of [FeCp*(dppe)Cl] in the presence of NH 4 PF 6 with 1,3,5-triethynylbenzene and with 1-bromo-3,5-bis(ethynyl)benzene, both followed by deprotonation with KOBu t , produced respectively the dendrons 1 and 2 . The hexanuclear compound 3 was obtained in two methods under Sonogashira reactions: (i) Sonogashira reaction between dendron 1 and 1,3,5-triiodobenzene catalysed by Pd(PPh 3 ) 2 Cl 2 and CuI and (ii) reaction of dendron 2 with 1,3,5-triethynylbenzene under the same conditions. Full size image The hexanuclear compound 3 was obtained as deep orange microcrystals using two methods shown in Fig. 1 : (i) Sonogashira reaction between dendron 1 and 1,3,5-triiodobenzene catalysed by [Pd(PPh 3 ) 2 Cl 2 ] and CuI ( Fig. 1 ) giving 3 with 50% yield and (ii) reaction of dendron 2 with 1,3,5-triethynylbenzene under the same conditions (55% yield). The 31 P NMR spectrum (C 6 D 6 ) of 3 exhibits a broad signal (99.39 δp.p.m.) due to the steric hindrance in the hexanuclear complex revealing slow rotation on the NMR timescale. The characterizations of the complex 3 are gathered in Supplementary Figs 13–18 . The dodecairon complex 4 was synthesized from the reaction between dendron 1 and hexakis(4-iodophenyl)-benzene catalysed by [Pd(PPh 3 ) 2 Cl 2 ] and CuI ( Fig. 2a ). Its infrared spectra show the disappearance of the absorption band around 2,275 cm −1 corresponding to the free alkynyl absorption ( ν C ≡ C ). The characterizations of the complex 4 are gathered in Supplementary Figs 19–24 . 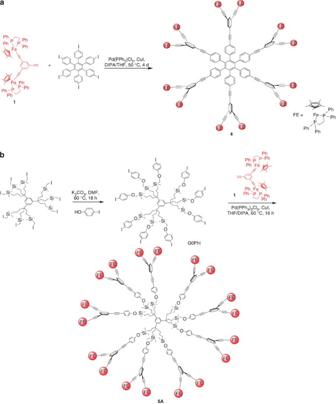Figure 2: Syntheses of dendrimers 4 and 5A by Sonogashira reactions. (a) The dodecairon complex4was synthesized from the Songashira reaction between dendron1and hexakis(4-iodophenyl)-benzene. (b) Thep.iodophenyl-terminated dendrimer with nine branches was synthesized from the dendritic core 1,3,5-{C[(CH2)3SiMe2CH2I]3}3-C6H3, G0-CH2I, by Williamson reaction withp.iodophenol. These dendritic precursors were then functionalized with dendron1according to Sonogashira reaction to give the dendrimer5A. Figure 2: Syntheses of dendrimers 4 and 5A by Sonogashira reactions. ( a ) The dodecairon complex 4 was synthesized from the Songashira reaction between dendron 1 and hexakis(4-iodophenyl)-benzene. ( b ) The p .iodophenyl-terminated dendrimer with nine branches was synthesized from the dendritic core 1,3,5-{C[(CH 2 ) 3 SiMe 2 CH 2 I] 3 } 3 -C 6 H 3 , G0-CH 2 I, by Williamson reaction with p .iodophenol. These dendritic precursors were then functionalized with dendron 1 according to Sonogashira reaction to give the dendrimer 5A . Full size image From the known dendritic cores 1,3,5{C[(CH 2 ) 3 SiMe 2 CH 2 I] 3 } 3 -C 6 H 3 , G0-CH 2 I, containing 9 terminal iodomethylsilyl branches ( Fig. 2b ), and the 27 iodomethylsilyl-terminated analogue G1-CH 2 I ( Fig. 3 ), azido- ( Figs. 4 and 5 ) and p .iodophenyl-terminated ( Figs 2 and 3 ) dendrimers were synthesized with 9 and 27 branches by I/N 3 substitution or Williamson reactions with p .iodophenol, respectively. These dendritic precursors were then functionalized with dendron 1 according to Sonogashira ( Figs 2 and 3 ) and ‘click’ reactions ( Figs 4 and 5 ), respectively. The characterizations of complexes G0-PhI and 5A are gathered in Supplementary Figs 25–27 and 28–33 , respectively. Those of complexes G1-PhI and 6A are gathered in Supplementary Figs 34–36 and 37–41 , respectively, and those of complexes 5B and 6B are gathered in Supplementary Figs 42–47 and 48–53 , respectively. 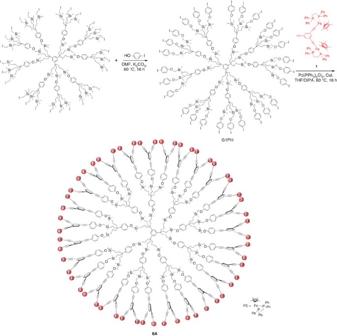Figure 3: Syntheses of dendrimer 6A by Sonogashira reaction. The dendrimer6Awas obtained under the identical strategies with dendrimer5Afrom 27 iodomethylsilyl-terminated analogue G1-CH2I. Figure 3: Syntheses of dendrimer 6A by Sonogashira reaction. The dendrimer 6A was obtained under the identical strategies with dendrimer 5A from 27 iodomethylsilyl-terminated analogue G1-CH 2 I. 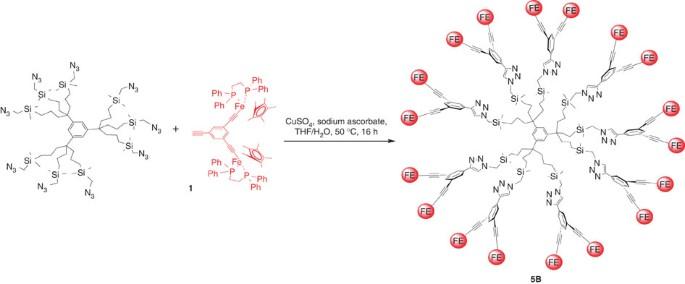Figure 4: Syntheses of dendrimer 5B by CuAAC ‘click’ reaction. Azido-dendrimer with nine branches was synthesized by I/N3substitution from the dendritic core 1,3,5-{C[(CH2)3SiMe2CH2I]3}3-C6H3, G0-CH2I, containing nine terminal iodomethylsilyl. This dendritic precursor was then functionalized with dendron1according to ‘click’ reaction to give the dendrimer5B. Full size image Figure 4: Syntheses of dendrimer 5B by CuAAC ‘click’ reaction. Azido-dendrimer with nine branches was synthesized by I/N 3 substitution from the dendritic core 1,3,5-{C[(CH 2 ) 3 SiMe 2 CH 2 I] 3 } 3 -C 6 H 3 , G0-CH 2 I, containing nine terminal iodomethylsilyl. This dendritic precursor was then functionalized with dendron 1 according to ‘click’ reaction to give the dendrimer 5B . 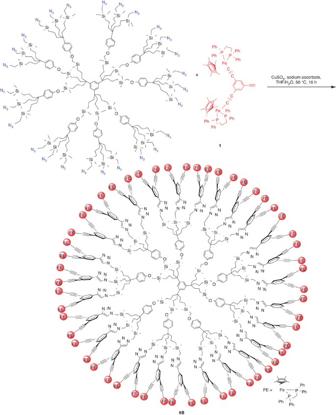Figure 5: Syntheses of dendrimer 6B by CuAAC `click' reaction. The dendrimer6Bwas obtained under the identical strategies with dendrimer5Bfrom 27 iodomethylsilyl-terminated analogue G1-CH2I. Full size image Figure 5: Syntheses of dendrimer 6B by CuAAC `click' reaction. The dendrimer 6B was obtained under the identical strategies with dendrimer 5B from 27 iodomethylsilyl-terminated analogue G1-CH 2 I. Full size image Diffusion-ordered spectroscopy experiments were carried out for the dendrimers 3 , 4 , 5A , 5B , 6A and 6B . The main goal was to determine the diffusion coefficient D leading to the hydrodynamic radii of the dendrimer. The spectra also reflected the purity of the products (the measurements were reproducible). The dendrimer size was found to regularly increase with the increase of the number of Fe(II) units at the dendrimer periphery. Also, the values obtained from dynamic light scattering (DLS) were much larger than the sizes obtained from diffusion-ordered spectroscopy and simulation owing to intermolecular associations [34] . The data are gathered in Table 1 . Table 1 Size parameters. Full size table The cyclic voltammograms of all the metallodendrons and metallodendrimers ( Supplementary Fig. 54 ) were recorded. They showed two reversible waves around −0.5 and −0.6 V, respectively, with a wave separation (Δ E p ) of 0.11–0.13 V for the metallodendrons ( Table 2 ) with a slight solvent effect and only around 0.070–0.080 V for the metallodendrimers. For the later, the cyclic voltammogram waves are broad with significant adsorption owing to their large size, which prevents clear wave separation and accuracy in the determination of the potentials, although the comproportionation constants ( Table 2 ) are sufficient for further syntheses of the mixed-valent complexes ( vide infra ). Table 2 Compared E 1/2 and comproportionation constant values. Full size table Synthesis of the oxidized metallodendrimers Mixed-valent complexes that are indicators of electronic communication between neighbouring redox sites [35] are useful tools and models of electronic communication in nanomaterials [36] . The neutral Fe II metallodendrimers 3 , 4 , 5B and 6B have been oxidized in dichloromethane (DCM) to the deep-blue fully oxidized (Fe III Fe III ) metallodendrimers 3 (PF 6 ) 6 , 4 (PF 6 ) 12 , 5B (PF 6 ) 18 , 6B (PF 6 ) 54 using one equiv. ferricinium hexafluorophosphate (FcH + PF 6 − ) per Fe centre. Oxidation to the green mixed-valent metallodendrimers 3 (PF 6 ) 3 , 4 (PF 6 ) 6 , 5B (PF 6 ) 9 and 6B (PF 6 ) 27 was conducted using only one equiv. FcH + PF 6 − per metallodendron. Alternatively, these mixed-valent metallodendrimers were synthesized on mixing equimolecular amounts of the Fe II metallodendrimers and the fully oxidized Fe III metallodendrimers ( Figs 6 and 7 ). Ferrocene that was formed in these reactions was removed on washing with pentane, and the oxidized metallodendrimers were characterized by Fourier transform infrared ( Supplementary Figs 55–70 and Supplementary Table 1 ), Mössbauer spectroscopies ( Supplementary Fig. 71 and Supplementary Table 2 ), near-infrared ( Supplementary Fig. 72 and Supplementary Table 3 ), ultraviolet–visible ( Supplementary Table 4 ) and elemental analysis. 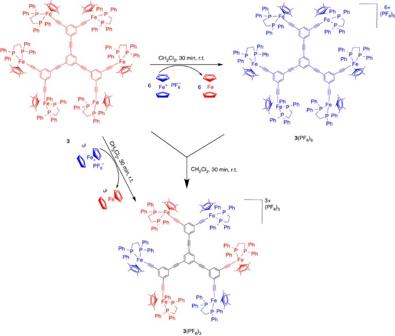Figure 6: Oxidation of metallodenrimers. Oxidation of the metallodendrimer3to the mixed-valent dendrimer3(PF6)3and fully oxidized dendrimer3(PF6)6. The FeIIspecies are in red and the FeIIIspecies are in blue. Figure 6: Oxidation of metallodenrimers. Oxidation of the metallodendrimer 3 to the mixed-valent dendrimer 3 (PF 6 ) 3 and fully oxidized dendrimer 3 (PF 6 ) 6 . The Fe II species are in red and the Fe III species are in blue. 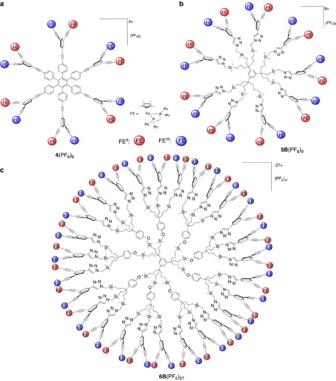Figure 7: Oxidation of metallodenrimers. (a–c) The following mixed-valent metallodendrimers4(PF6),5B(PF6)9and6B(PF6)27have been obtained analogously. The FeIIspecies are in red and the FeIIIspecies are in blue. Full size image Figure 7: Oxidation of metallodenrimers. ( a – c ) The following mixed-valent metallodendrimers 4 (PF 6 ), 5B (PF 6 ) 9 and 6B (PF 6 ) 27 have been obtained analogously. The Fe II species are in red and the Fe III species are in blue. Full size image The infrared spectra of all the multinuclear iron(II) and iron(III) complexes display a single C≡C stretching band around 2,040 and 2,000 cm −1 , respectively ( Supplementary Table 1 ). In contrast, the infrared spectra of all the mixed-valent complexes show two distinct C≡C stretching bands at these wavenumbers, providing evidence for localized oxidation states at 10 13 s −1 . The Mössbauer spectra of all the mixed-valent complexes recorded at 78 K show two quadrupole doublets of approximately equal intensities corresponding to the Fe II and Fe III states ( Supplementary Table 2 ), indicating localized mixed valency at 10 −7 s −1 . The intervalence charge transfer (IVCT) band ( Supplementary Table 3 ) of the four mixed-valent complexes was found in the near-infrared region in CD 3 COCD 3 . The full width at half height of the band is very close to the theoretical value derived from the near-infrared band position λ max according to Hush’s relationship for symmetrical mixed-valent complexes. The ratios (Δ ν 1/2 ) obs /(Δ ν 1/2 ) calc were less than 1.15, falling in the 1.1–1.4 range of class-II mixed-valent complexes [36] , [37] , [38] . The UV-vis spectra of all the multinuclear complexes ( Supplementary Table 4 ) display intense absorption bands in the range 250–380 nm (LC π–π* transition) and around 400 nm (metal to ligand charge transfer (MLCT) transition) responsible for the orange colour of the neutral compounds and also present in the deep colour of the mixed-valent/fully oxidized products, whereas the oxidized complexes present two transitions above 550–580 and 645–680 nm explaining their green/blue colour [38] . The mixed-valent properties of all the mixed-valent dendrimers are further discussed in the Supplementary Notes 1–5 . Stabilization of AuNPs The availability of metallodendrimers in three oxidation states with 54 Cp*Fe(dppe)alkynyl termini with interiors containing or not 1,2,3-triazole ligands offered the opportunity to examine the influence of the intradendritic presence of these triazole ligands on the stabilization of AuNPs [39] , [40] , [41] , [42] . Indeed, it was possible to start either from Fe II Fe II metallodendrimers to reduce Au III into AuNPs (equation (1)) or from Fe III Fe III metallodendrimers and Au III and to reduce the mixture using excess NaBH 4 to Fe II Fe II and AuNPs (equation (2)). These experiments were conducted with the dendrimer 6A and 6B and with dendron 1 for comparison, and the results are gathered in Table 3 and Supplementary Figs 73–82 . Table 3 Properties of AuNPs prepared by the methods of equations (1) and (2). Full size table The AuNPs formed from 6A gave a much more intense plasmon absorption in the ultraviolet–visible spectrum than 6B around 530 nm indicating much larger AuNPs ( Fig. 8 ). Accordingly, the smallest AuNPs (cores: 1.4 and 1.9 nm from equation (1) resp. equation (2)) were obtained with the ‘click’ metallodendrimer 6B . The Sonogashira metallodendrimer 6A gave larger AuNPs (cores: 3.4 and 3.7 nm from equation (1) resp. equation (2)), and the metallodendron 1 gave large AuNPs with equation (1) (20 nm core), but small AuNPs (2 nm core) according to equation (2) ( Fig. 9 ). 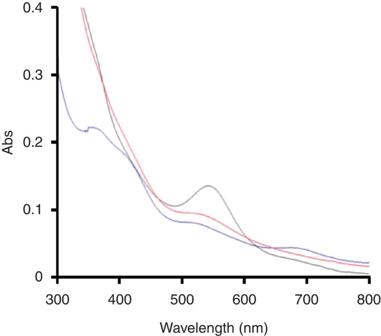Figure 8: Compared ultraviolet–visible absorption spectra in CH2Cl2. The AuNPs stabilized by reaction of NaBH4with a mixture of HAuCl4and dendron1[PF6]2(blue line),6A[PF6]54(black line) or6B[PF6]54(red line) under identical conditions giving back the neutral dendrimers (equation (2)). Figure 8: Compared ultraviolet–visible absorption spectra in CH 2 Cl 2 . The AuNPs stabilized by reaction of NaBH 4 with a mixture of HAuCl 4 and dendron 1 [PF 6 ] 2 (blue line), 6A [PF 6 ] 54 (black line) or 6B [PF 6 ] 54 (red line) under identical conditions giving back the neutral dendrimers (equation (2)). 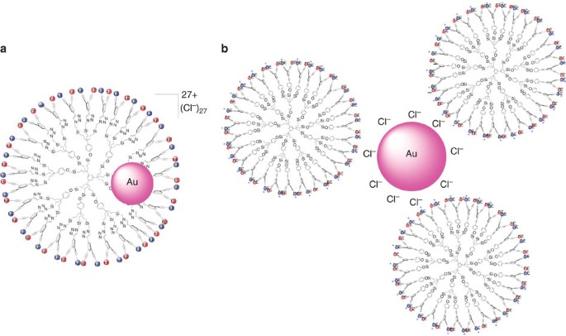Figure 9: Schematic picture representing the AuNP stabilized by dendrimers. (a) Intradendritic AuNP stabilization by a ‘click’ dendrimer6B27+involving AuNP-triazole interactions. (b) Interdendritic stabilization by many ‘Sonogashira’ dendrimers6A27+. It is likely that chloride anions surround the AuNPs in both cases. Full size image Figure 9: Schematic picture representing the AuNP stabilized by dendrimers. ( a ) Intradendritic AuNP stabilization by a ‘click’ dendrimer 6B 27+ involving AuNP-triazole interactions. ( b ) Interdendritic stabilization by many ‘Sonogashira’ dendrimers 6A 27+ . It is likely that chloride anions surround the AuNPs in both cases. Full size image In this work, the syntheses and characterizations of metallodendrimers in three oxidation states have been achieved for the first time, allowing redox interplay exemplified by the formation of AuNPs of selective size depending on the presence and number of intradendritic 1,2,3-triazole ligands. The metallodendrimers have been designed using interacting metal centres in new bimetallic dendrons. It is the electronic communication between these two iron centres within each bimetallic dendron that provides the occurrence of another stable oxidation state that is class-II mixed-valent in the Robin–Day classification as shown by the splitting of the C≡C stretching band in infrared and presence of a near-infrared intervalent band. The choice of the method of dendron connection to dendrimer cores, Sonogashira versus ‘click’ reaction, further results in the presence or absence of ‘clicked’ 1,2,3-triazolyl intradendritic ligands. This dendrimer engineering providing electronic flexibility is unique in that the stability and isolation of different dendrimer oxidation states allow examining the influence of the presence and number of these triazole ligands on the intradendritic coordination of Au III moieties. As a consequence, it could be shown here that the intradendritic AuNP stabilization specifically induces the formation of small AuNPs. The results are well taken into account by coordination of Au 3+ by the triazole ring in both equations (1) and (2) experiments followed by reduction to small monodisperse AuNPs (1.4±0.3 nm) having a core size slightly higher than 27 Au atoms inside a dendrimer, owing to some leaching of Au atoms among dendrimers (the diameter of a 27-atom AuNP is 1 nm). The triazole loosely interacts with the AuNP surface, which contributes to its intradendritic stabilization of these small AuNPs. On the contrary, the larger AuNPs stabilized by the Sonagashira dendrimer 6B gather a number of atoms around 1,400, which involves considerable distribution around dendrimer peripheries and final stabilization of each AuNP by several dendrimers, because Au III reduction essentially proceeds outside dendrimers, and there are no heteroatom-containing ligand retaining AuNPs inside the dendrimers ( Fig. 10 ). The small dendrons allow the formation of a very large AuNP core surrounded by a large number of dendrons because small dendrons are much less efficient than large dendrimers for NP stabilization. 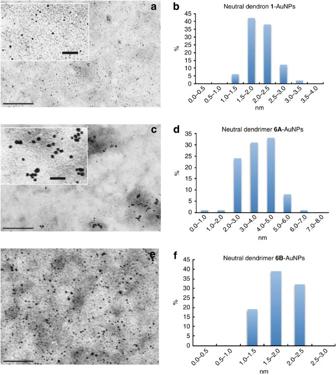Figure 10: Transmission electron microscopy of AuNPs. AuNPs stabilized by reaction of NaBH4 with a mixture of HAuCl4and dendron1[PF6]2(aandb),6A[PF6]54(candd) or6B[PF6]54(eandf) under identical conditions giving back the neutral dendrimers. Scale bars;aandc, 100nm:a(inset) andc(inset), 20 nm;e, 50 nm.. Figure 10: Transmission electron microscopy of AuNPs. AuNPs stabilized by reaction of NaBH4 with a mixture of HAuCl 4 and dendron 1 [PF 6 ] 2 ( a and b ), 6A [PF 6 ] 54 ( c and d ) or 6B [PF 6 ] 54 ( e and f ) under identical conditions giving back the neutral dendrimers. Scale bars; a and c , 100nm: a (inset) and c (inset), 20 nm; e , 50 nm.. Full size image Remarkably, the AuNP core size of the Au III -‘click’-dendrimer complexes does not vary considerably with the mode of formation for the dendrimers 6A and 6B whatever the synthetic route (equation (1) versus equation (2)). Indeed, the AuNP core size approximately corresponds to the number of Au atoms generated from the triazolyl-coordinated Au III precursors in a single dendrimer. It does for dendron 1 , however, because AuNP stabilization by borohydride then predominates in equation (2) in the absence of strong dendritic stabilization. On the other hand, the related non-‘click’ (Sonogashira) dendrimers generate much larger AuNPs formed outside the metallodendrimers, but also stabilized by a group of metallodendrimers around the AuNP ( Supplementary Notes 6 and 7 ). Such a nanomaterial engineering strategy should be most useful for the design of sophisticated nanosensors, nanocatalysts, nanobatteries and nanopolyelectrolytes in the near future [6] . Synthesis and characterizations of dendron 1 1,3,5-Triethynylbenzene (150 mg, 1 mmol) in 10 ml distilled THF was added to a solution of [FeCp*(dppe)Cl] (1.56 g, 2.5 mmol) and NH 4 PF 6 (326 mg, 2 mmol) in 12 ml CH 3 OH. The suspension was stirred at room temperature (r.t.) for 16 h. The solvent was evaporated in vacuo . The residual solid was dissolved in 5 ml distilled DCM, 100 ml distilled pentane was added and the precipitation was washed with pentane for another two times. The residual solid was dissolved in 10 ml distilled THF, and then potassium tert -butoxide (224 mg, 2 mmol) was added in a single portion. The mixture was stirred 3 h under r.t., the solvent was removed in vacuo and the residue was extracted with distilled diethylether to form the crude compound that was further purified by column chromatography (pentane/diethylether=5/1, R f =0.2) providing dendron 1 as an orange powder (795.6 mg, yield=60%). Matrix-assisted laser desorption/ionization time of flight (MALDI-TOF): calc. m / z for M + (C 84 H 82 Fe 2 P 4 ) 1,327.1, found 1,326.4. Anal. calcd. for C 84 H 82 Fe 2 P 4 : C, 76.02; H, 6.23. Found: C, 76.32; H, 6.38. For dendron 2 , a similar procedure was used. See Supplementary Methods for remaining syntheses; full characterization of all other complexes are not described herein. Synthesis of dendrimer 6A using a Sonogashira reaction A mixture of dendron 1 (121 mg, 1.5 equiv. for each branch), G1-PhI (25 mg, 1 equiv. for each branch) and catalytic amount of Pd(PPh 3 ) 2 Cl 2 (8.5 mg, 0.2 equiv. for each branch) and CuI (4.6 mg, 0.1 equiv. for each branch) were dissolved in the mixed solvent of distilled diisopropylamine (DIPA)/THF 10 ml. The solution was stirred overnight at 50 °C under N 2 . The solvent was evaporated in vacuo . The residual solid was extracted with PhCH 3 30 ml, the solution was dried with anhydrous Na 2 SO 4 , the solvent was removed in vacuo and the dark red residue was washed three times with distilled diethyl ether 50 ml to remove the excess free ligand. Then the residual solid was dissolved in 1 ml of dry THF, 100 ml of dry CH 3 CN was added to the mixture and compound 6A precipitated as a deep orange solid (66 mg, yield=70%). Anal. calcd. for C 2718 H 2838 Fe 54 P 108 Si 36 O 36 : C, 75.13; H, 6.58. Found: C, 75.44; H, 6.47. Synthesis of dendrimer 6B by ‘click’ reaction To a mixture of G1-N 3 (20 mg, 3.6 × 10 −3 mmol, 1 equiv.) and dendron 1 (193 mg, 0.146 mmol, 1.5 equiv. for each branch) in THF 20 ml, 10 ml of distilled H 2 O was added dropwise, and a solution of CuSO 4 ·5 H 2 O (36.5 mg, 0.146 mmol, 1.5 equiv. for each branch) in 1 ml of H 2 O was slowly added to the mixture at 0 °C, which provoked a colour change from orange to dark brown. The solution of sodium ascorbate (57.8 mg, 0.292 mmol, 3 equiv. for each branch) was dropwise added to this mixture at 0 °C, which resulted in a colour change from dark brown to orange. Stirring was continued at 50 °C under N 2 for another 16 h, the solvent was evaporated in vacuo until only the aqueous phase was left, 50 ml of toluene, 50 ml of H 2 O and 3 ml of ammonium hydroxide was added to the solution and the mixture was stirred at r.t. for 30 min for extraction of the Cu catalyst. After separation, the organic phase was dried with anhydrous Na 2 SO 4 , and the solvent was removed in vacuo , which gave a deep orange solid that was washed three times with 300 ml diethyl ether to remove the excess free ligands. This procedure yielded the ‘click’ dendrimer as an orange solid (89.2 mg, 60%). Anal. calcd. for C 2556 H 2757 Fe 54 P 108 N 81 O 9 Si 36 : C, 72.87; H, 6.60; N, 2.69. Found: C, 72.69; H, 6.40; N, 2.45. The synthesis and characterizations of 5B were conducted under similar conditions. Oxidation of the complex 6B to 6B (PF 6 ) 27 The dendrimer 6B (82 mg, 2 × 10 −3 mmol, 1 equiv.) was dissolved in 5 ml distilled DCM, and [FeCp 2 ] [PF 6 ] (17.7 mg, 0.0535, mmol, 27 equiv.) was added in a single portion to this solution at r.t., which provoked an immediate colour change from orange to dark green, the solution was stirred for 4 h at r.t. under N 2 , the solvent was removed in vacuo until 0.5 ml was left, then 50 ml of distilled pentane was added to this dark green solution and the mixed-valent dendrimer was precipitated. After filtration, the residual solid was washed twice more with 100 ml pentane, and the residue was dried under vacuum to give the mixed-valent dendrimer as a dark solid (80.9 mg, 90% yield. Anal. calcd. for C 2556 H 2757 Fe 54 P 108 N 81 O 9 Si 36 (PF 6 ) 27 : C, 66.68; H, 6.04; N, 2.46. Found: C, 66.77; H, 6.20; N, 2.45. The oxidation of 3, 4, 5B and 6B by [FeCp 2 ] [PF 6 ] to the mixed-valent or fully oxidized dendrimers were conducted identically. Synthesis of AuNPs stabilized by dendrimer 6B 27+ The neutral dendrimer 6B (10 mg, 2.419 × 10 −4 mmol, 1 equiv. per branch) was dissolved in 2 ml DCM, and the solution of HAuCl 4 (0.86 mg, 2.175 × 10 −3 mmol, 1/3 equiv.) in 2 ml of acetone was slowly added to the mixture at r.t., which provoked a colour change from orange to deep green. Stirring was continued for another 30 min. Infrared (KBr): 2,036 cm −1 ( ν C≡C-Fe(II) ), 2,009 cm −1 ( ν C≡C-Fe(III) ). Ultraviolet–visible: λ max 1 =410 nm (ν Π-Π* ), λ max 2 / λ max 3 =580/665 nm (ν LMCT ). Transmission electron microscopy: 1.4±0.3 nm. The synthesis and characterizations of AuNPs stabilized by ionic mixed-valent dendron 1 + or dendrimer 6A 27+ were analogous. Synthesis of AuNPs stabilized by neutral dendrimer 6B The neutral dendrimer 6B (5 mg, 1.15 × 10 −4 mmol, 1 equiv.) was dissolved in 2 ml of DCM, and [FeCp 2 ] [PF 6 ] (2.1 mg, 6.22 × 10 −3 mmol, 54 equiv) was added under stirring, which resulted in an instantaneous colour change from orange to deep blue, and the mixture was stirred at r.t. during 4 h. Then, the solvent was removed in vacuo until 0.5 ml was left, 50 ml of distilled pentane was added to the mixture and the fully oxidized complex precipitated as a dark product. After filtration, this solid was dried under vacuum, dissolved in 2 ml of distilled DCM and a solution of HAuCl 4 (1 mg, 2.54 × 10 −3 mmol) in 2 ml methanol was added to the mixture under stirring, forming a blue solution. Then, a solution of NaBH 4 (2.35 mg, 6.2 × 10 −2 mmol, three equiv.) in 1 ml methanol was added dropwise under stirring, leading to a colour change from dark blue to deep violet, which indicated the formation of the AuNPs. The mixture was stirred at r.t. for another 10 min. Infrared (KBr): 2,045 cm −1 ( ν C≡C-Fe(II) ). Ultraviolet–visible: λ max 1 =410 nm ( ν Π-Π* ), λ max 2 =545 nm (plasmon band). Transmission electron microscopy: 1.9±0.3 nm. The synthesis and characterizations of AuNPs stabilized by the neutral dendron 1 or the dendrimer 6A were conducted analogously. How to cite this article: Wang, Y. et al. Metallodendrimers in three oxidation states with electronically interacting metals and stabilization of size-selected gold nanoparticles. Nat. Commun. 5:3489 doi: 10.1038/ncomms4489 (2014).